MicroRNA-30c inhibits human breast tumour chemotherapy resistance by regulating TWF1 and IL-11 Chemotherapy resistance frequently drives tumour progression. However, the underlying molecular mechanisms are poorly characterized. Epithelial-to-mesenchymal transition has been shown to correlate with therapy resistance, but the functional link and signalling pathways remain to be elucidated. Here we report that microRNA-30c, a human breast tumour prognostic marker, has a pivotal role in chemoresistance by a direct targeting of the actin-binding protein twinfilin 1, which promotes epithelial-to-mesenchymal transition. An interleukin-6 family member, interleukin-11 is identified as a secondary target of twinfilin 1 in the microRNA-30c signalling pathway. Expression of microRNA-30c inversely correlates with interleukin-11 expression in primary breast tumours and low interleukin-11 correlates with relapse-free survival in breast cancer patients. Our study demonstrates that microRNA-30c is transcriptionally regulated by GATA3 in breast tumours. Identification of a novel microRNA-mediated pathway that regulates chemoresistance in breast cancer will facilitate the development of novel therapeutic strategies. Therapy resistance, whether intrinsic or acquired, is one of the most fundamental problems in cancer, and contributes to local and distant tumour recurrence and disease progression. A better understanding of the underlying molecular mechanisms will undoubtedly lead to the development of more effective therapies. Non-coding single-stranded microRNAs (miRNAs, miRs) have emerged as important epigenetic regulators of protein-coding genes and aberrant miRNA expression has been found in many cancers [1] . However, the role of miRNAs in chemoresistance remains to be characterized. In addition, the epithelial-to-mesenchymal transition (EMT) has been connected to breast cancer chemoresistance [2] , [3] , but the regulatory link is unknown. We therefore hypothesized that miRNAs that regulate EMT might be critical for regulating drug resistance. The miRNAs inhibit target genes primarily by degrading mRNA or by repressing translation via seed sequence-mediated imperfect complementary binding to 3′ untranslated regions (3′UTRs) [4] , [5] . By combining microarray analyses, miRNA target prediction algorithms and experimental validation approaches, we sought to identify miRNA targets that regulate EMT and drug resistance in breast cancer cells. miR-30c is a prognostic biomarker in breast cancer To identify miRNA biomarkers, we profiled primary breast tumour miRNA expression levels and performed clinicopathological correlation analyses for breast tumours collected under Institutional Review Board-approved protocols at the University of Chicago Breast SPORE and in independent data sets. Frozen primary breast tumour tissues (University of Chicago (UC) tumour set, n =46) and adjacent normal tissues ( n =5) were first profiled for both gene and miRNA expression. Of 757 expressed miRNAs, 152 passed the filtering criteria for subsequent unsupervised hierarchical clustering ( Fig. 1a ; see also patient information in Supplementary Table S1 ). Unsupervised clustering divided the miRNAs into cluster A and cluster B, and these miRNAs displayed distinct expression patterns in the UC breast tumour set. Specifically, cluster A miRNAs were upregulated in group one tumours and cluster B miRNAs were upregulated in group two tumours. 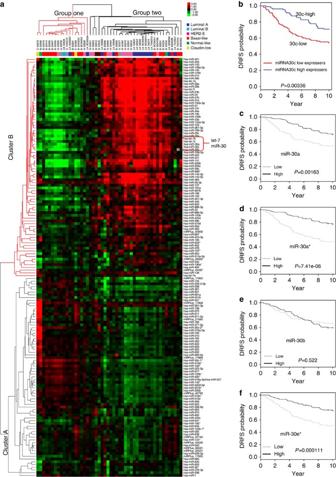Figure 1: miRNA profiling of humRNAs and breast tumour samples. (a) Heat map diagram with two-way unsupervised hierarchical clustering of miRNAs and breast tumour samples. Each row represents an miRNA and each column represents a sample. The miRNA clustering tree is shown on the left (cluster A and B), and the sample clustering tree appears at the top (group one and two). The colour scale shown in the map illustrates the relative expression level of a miRNA across all samples: red represents an expression level above the mean; green represents expression lower than the mean. Black means median expression. Levels of 152 miRNAs passed filtering and shown from 51 frozen human breast samples (46 breast tumours and 5 normal mammary tissues). NL-normal-like, LA-luminal A, LB-luminal B, B-basal-like, H-HER2-enriched, C-claudin-low, U-undetermined, N-normal (normal breast tissue adjacent to tumours). (b–f) Kaplan–Meier plots of distant relapse-free survival (DRFS) based on the expression of miR-30 family members (30c, 30a, 30a*, 30b and 30e*). Associations of miR-30 members with DRFS were analysed with GSE22216 breast cancer data set (n=210) deposited by Buffaet al.6To define low (blue) and high (red) expressers, samples were rank-ordered based on miRNA30 expression and the top 50% samples were defined as high expressers. Log rank testP-values are shown. Figure 1: miRNA profiling of humRNAs and breast tumour samples. ( a ) Heat map diagram with two-way unsupervised hierarchical clustering of miRNAs and breast tumour samples. Each row represents an miRNA and each column represents a sample. The miRNA clustering tree is shown on the left (cluster A and B), and the sample clustering tree appears at the top (group one and two). The colour scale shown in the map illustrates the relative expression level of a miRNA across all samples: red represents an expression level above the mean; green represents expression lower than the mean. Black means median expression. Levels of 152 miRNAs passed filtering and shown from 51 frozen human breast samples (46 breast tumours and 5 normal mammary tissues). NL-normal-like, LA-luminal A, LB-luminal B, B-basal-like, H-HER2-enriched, C-claudin-low, U-undetermined, N-normal (normal breast tissue adjacent to tumours). ( b – f ) Kaplan–Meier plots of distant relapse-free survival (DRFS) based on the expression of miR-30 family members (30c, 30a, 30a*, 30b and 30e*). Associations of miR-30 members with DRFS were analysed with GSE22216 breast cancer data set ( n =210) deposited by Buffa et al . [6] To define low (blue) and high (red) expressers, samples were rank-ordered based on miRNA30 expression and the top 50% samples were defined as high expressers. Log rank test P -values are shown. Full size image The hsa-miR-30 family segregated with the cluster B miRNAs with high expression in group two patient tumours, including many known tumour-suppressor miRs, such as the let-7 family members ( Fig. 1a ). To determine the role of the miR-30 family members in breast cancer progression, we first examined their clinical relevance for patient survival. In an independent Oxford breast tumour data set containing a retrospective series of 10-year follow-up cases ( n =210) with matched miRNA and mRNA expression arrays (GSE 22216 and GSE22220, respectively) [6] , we identified miR-30c as well as miR-30a, -30a* and -30e* as individual favourable breast cancer prognostic markers for distant relapse-free survival (DRFS; Fig. 1b ). The prognostic role of miR-30c is still significant even when adjusted for age, tumour size, oestrogen receptor (ER) status, nodal status and histological grade ( Supplementary Table S2 ). Furthermore, when breast tumour subtypes are classified based on the PAM50 subtype predictor [7] and the nine cell line claudin-low predictor [8] , miR-30c expression is associated with breast tumour subtypes in two independent data sets (UC tumour set and Oxford tumour set [6] ; Supplementary Fig. S1a-c ) and its prognostic role is subtype-dependent ( Supplementary Table S3 ). However, the miR-30c levels were not significantly different between paired primary breast tumours and normal breast tissue adjacent to tumours ( Supplementary Table S4 ). By univariate analysis of a previous report, both miR-30a* and miR-30c have been shown to correlate with the benefit of tamoxifen treatment and longer progression-free survival in oestrogen receptor (ER)-positive breast cancer patients [9] . However, in that study miR-30c was the only independent miRNA predictor of tamoxifen treatment response by multivariate analysis when adjusted for other clinico-phathological factors [9] . We hypothesized that the miR-30 family, especially miR-30c, might functionally regulate therapy response in addition to having an association with treatment benefits. We therefore focused on their role in chemoresistance regulation in breast cancer. miR-30c regulates chemoresistance of breast cancer cells To test our hypothesis that miR-30c has a role in breast tumour progression and chemoresistance, we investigated the relevance of miR-30c to chemotherapy-induced cytotoxicity of tumour cells. Interestingly, for six breast cancer cell lines (T47D, MCF-7, MDA-MB-231, BT-20, HCC-70 and HCC-38), we observed a significant inverse correlation between miR-30c levels and cell survival in response to paclitaxel (0.1–50 nM) and doxorubicin (1–500 nM) treatments, represented as Log2-transformed expression levels and AUC (the area under the survival curve, in a series of six treatment doses; Fig. 2a , P =0.04). These correlations are more significant at the highest doses of paclitaxel (50 nM) and doxorubicin (500 nM) ( Supplementary Fig. S2a,b and Supplementary Table S5 , P =0.0198 and 0.0191, respectively). 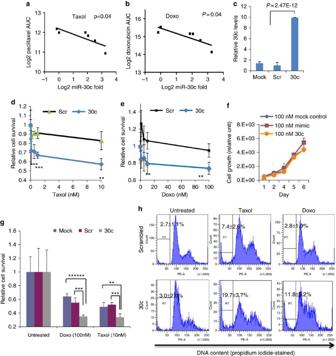Figure 2: miR-30c corresponds to and regulates chemoresistance of breast cancer cells. (a-b) Association of Log2-transformed miR-30c expression (fold) with the survival (log2-transformed AUC) of breast cancer cell lines (n=6, T47D, MCF-7, MDA-MB-231, BT20, HCC70 and HCC38) in response to paclitaxel (Taxol) at 0.1–50 nM (a) and doxorubicin at 1–500 nM (b). A linear correlation testP=0.04 for both association studies. (c) Log2-transformed expression levels of miR-30c in MDA-MB-231 cells 48 h after oligo transfections, measured by real-time PCR.P=2.47E-12 by a Student’st-test (n=3). Error bars represent the s.d. of the mean. (d,e) Cell survival of MDA-MB-231 cells after transient transfection of scrambled control and mature miR-30c oligos, upon 72-h exposure to different doses of paclitaxel (Taxol,d) and doxorubicin (Doxo,e). Student’st-testP=0.00022 (0.5 nM), 0.00014 (1.0 nM) and 0.00191 (10 nM) for Taxol treatment, andP=0.00802 (10 nM) and 0.00212 (100 nM) for Doxo treatment, comparing 30c samples with Scr samples (n=6). Error bars: s.d.(f) No significant effect of transient transfection of miR-30c on the growth rate of MDA-MD-231 cells, compared with a mock transfection control and a scrambled RNA mimic control. Error bars: s.d. (g) miR-30c sensitized the drug response of BT-20 breast cancer cells to 48-h treatment of doxorubicin (100 nM) and paclitaxel (Taxol, 10 nM). When comparing 30c with controls, Student’st-testP=5.52E-07 (mock) and 0.0003 (Scr) for Doxo,P=0.0066 (mock) and 0.0009 (Scr) for Taxol (n=5). Error bars: s.d. (h) Representative flow profiles of BT20 breast cancer cell DNA content upon 24-h treatment of paclitaxel (Taxol, 10 nM) or doxorubicin (Doxo, 100 nM). The gated sub-G1 population represents early apoptotic cells. The s.d. values of the mean are shown. Figure 2: miR-30c corresponds to and regulates chemoresistance of breast cancer cells. ( a - b ) Association of Log2-transformed miR-30c expression (fold) with the survival (log2-transformed AUC) of breast cancer cell lines ( n =6, T47D, MCF-7, MDA-MB-231, BT20, HCC70 and HCC38) in response to paclitaxel (Taxol) at 0.1–50 nM ( a ) and doxorubicin at 1–500 nM ( b ). A linear correlation test P =0.04 for both association studies. ( c ) Log2-transformed expression levels of miR-30c in MDA-MB-231 cells 48 h after oligo transfections, measured by real-time PCR. P =2.47E-12 by a Student’s t -test ( n =3). Error bars represent the s.d. of the mean. ( d , e ) Cell survival of MDA-MB-231 cells after transient transfection of scrambled control and mature miR-30c oligos, upon 72-h exposure to different doses of paclitaxel (Taxol, d ) and doxorubicin (Doxo, e ). Student’s t -test P =0.00022 (0.5 nM), 0.00014 (1.0 nM) and 0.00191 (10 nM) for Taxol treatment, and P =0.00802 (10 nM) and 0.00212 (100 nM) for Doxo treatment, comparing 30c samples with Scr samples ( n =6). Error bars: s.d. ( f ) No significant effect of transient transfection of miR-30c on the growth rate of MDA-MD-231 cells, compared with a mock transfection control and a scrambled RNA mimic control. Error bars: s.d. ( g ) miR-30c sensitized the drug response of BT-20 breast cancer cells to 48-h treatment of doxorubicin (100 nM) and paclitaxel (Taxol, 10 nM). When comparing 30c with controls, Student’s t -test P =5.52E-07 (mock) and 0.0003 (Scr) for Doxo, P =0.0066 (mock) and 0.0009 (Scr) for Taxol ( n =5). Error bars: s.d. ( h ) Representative flow profiles of BT20 breast cancer cell DNA content upon 24-h treatment of paclitaxel (Taxol, 10 nM) or doxorubicin (Doxo, 100 nM). The gated sub-G1 population represents early apoptotic cells. The s.d. values of the mean are shown. Full size image We further characterized the role of miR-30c in regulating chemotherapy resistance by modulating its levels in breast cancer cells. Transient transfection of miR-30c resulted in a significant decrease in survival of chemoresistant MDA-MB-231 breast cancer cells to paclitaxel (taxol, 0.5–10 nM) and doxorubicin (10–100 nM) at even low doses ( Fig. 2c–e ). Growth curve analyses suggested that increased miR-30c levels did not affect cancer cell growth ( Fig. 2f ). Elevated miR-30c also sensitized the drug response of a second breast cancer cell line BT-20 to paclitaxel and doxorubicin ( Fig. 2g ). Furthermore, DNA content analysis confirmed that miR-30c significantly increased the apoptotic sub-G1 population of these cancer cells upon paclitaxel and doxorubicin treatments ( Fig. 2h ). We also examined the effects of two other individual favourable breast cancer prognostic markers in the miR-30 family, miR-30a and -30a*, on the response of MDA-MB-231 breast cancer cells to chemotherapy drugs. Although ectopic miR-30a did not show any effect on doxorubicin treatment at various doses up to 200 nM, it did decrease breast cancer cell survival in response to paclitaxel at very high doses (50 nM; Supplementary Fig. S3a,b ). In addition, miR-30a* sensitized the drug response of breast cancer cells to doxorubicin (200 nM) and paclitaxel (5–50 nM) at relatively high doses ( Supplementary Fig. S3a,b ). miR-30c regulates EMT and targets cytoskeleton gene TWF1 To examine the molecular mechanisms by which miR-30c regulates chemoresistance, we investigated its target genes and focused on a few that relate to EMT regulation and cancer progression. Mammalian miRNAs regulate target genes primarily by decreasing mRNA levels [10] . Multiple computational algorithms, such as GeneSet2miRNA, which identifies miRNA activities by at least 4 of 11 established miRNA target prediction programmes [11] , can predict potential interactions between genes and miRNAs. To strategically identify direct miR-30c target genes, we used global transcriptome analysis (microarray) in combination with GeneSet2miRNA and experimental validation analyses, including immunoblots, luciferase assays and functional rescue studies. We first performed microarray analyses of MDA-MB-231 cells that were transiently transfected either with miR-30c oligos or the scrambled control. High miR-30c levels significantly inhibited the expression levels of 291 genes in many networks and pathways, such as anti-apoptosis and cytoskeleton genes ( Fig. 3a ; see also Supplementary Data 1 ). Using this list, we performed online GeneSet2miRNA [11] target gene prediction analysis and narrowed the direct targets of miR-30c down to 77 potential genes, predicted by a minimum of 4 out of 11 established algorithms ( Fig. 3a ; see also Supplementary Table S6 ). Among these, the cytoskeleton genes twinfilin 1 ( TWF1 , also known as PTK9 ) and vimentin ( VIM ) were reported to regulate cell motility, drug sensitivity and cancer progression [2] , [12] , [13] , [14] , [15] . 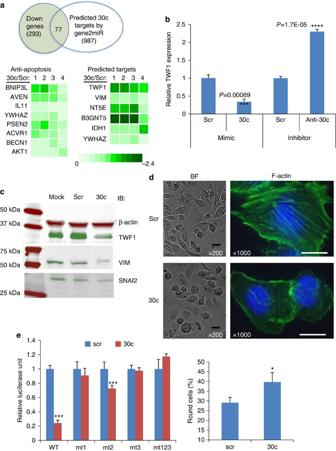Figure 3: miR-30c regulates EMT and directly targets TWF1. (a) Genes suppressed by miR-30c in breast cancer cells. Top panel: left circle shows the microarray data of 293 genes significantly inhibited by miR-30c in MDA-MB-231 cells (seeSupplementary Table S2). The right circle indicates the genes predicted as direct targets of miR-30c by Geneset2miR (by ≥4 of 11 algorithms) and overlapped genes are 77 (Supplementary Table S3). Bottom left panel: heatmap for eight anti-apoptotic genes inhibited by miR-30c. Bottom right panel: heatmap for predicted direct targets, downregulated in miR-30c-transfected cells. Green boxes are colour-coded based on log2-transformed expression reduction levels for four pairs of 30c/scrambled microarray comparisons. (b) Expression levels of TWF1 (measured by real-time PCR) upon transfection of miR-30c or the anti-miR-30c inhibitors into MDA-MB-231 cells. Student’st-testP-values are shown (n=3). Error bars: s.d. (c) Immunoblots of TWF1 (green band, top panel), VIM (green band, middle panel), SNAI2 (green band, bottom panel) and β-actin (red band, top panel) with protein lysates of MDA-MB-231 cells 36 h after transfections of mock control, scrambled (Scr) and oligo miRNA-30c, respectively. (d) Effects of miR-30c on cell morphology and F-actin. Top panels: images of MDA-MB-231 cells after miR-30c transfections. Top left panels: bright field (BF) images of cells (X200, black scale bars, 10 μm). Top right panels: fluorescent images (X1,000, white scale bars, 5 μm) with F-actin staining (green) and DAPI staining of DNA (blue). Bottom histogram: percentage of round cells counted in two groups, scrambled and 30c-transfected cells (n=4, counting 4 replicates of 100–150 cells). Cells were collected 36 h after transfections of scramble control (top) or miR-30c oligos (bottom). Student’st-testP=0.043. Error bars: s.d. (e) Luciferase activity assays of Hek293T cells co-transfected with miR-30c (or scrambled control, scr) and the luciferase vector containing wild-type (WT) or mutated (mt) 3′UTR of TWF1. Mt1, 2, 3 are mutants with G/C converted to T in individual predicted binding site 1, 2, or 3, and mt123 contains all three mutated sites (seeSupplementary Fig. S3). Student’st-testP=0.0001 for WT or mt2, comparing 30c with scr control (n=5). Error bars: s.d. Figure 3: miR-30c regulates EMT and directly targets TWF1. ( a ) Genes suppressed by miR-30c in breast cancer cells. Top panel: left circle shows the microarray data of 293 genes significantly inhibited by miR-30c in MDA-MB-231 cells (see Supplementary Table S2 ). The right circle indicates the genes predicted as direct targets of miR-30c by Geneset2miR (by ≥4 of 11 algorithms) and overlapped genes are 77 ( Supplementary Table S3 ). Bottom left panel: heatmap for eight anti-apoptotic genes inhibited by miR-30c. Bottom right panel: heatmap for predicted direct targets, downregulated in miR-30c-transfected cells. Green boxes are colour-coded based on log2-transformed expression reduction levels for four pairs of 30c/scrambled microarray comparisons. ( b ) Expression levels of TWF1 (measured by real-time PCR) upon transfection of miR-30c or the anti-miR-30c inhibitors into MDA-MB-231 cells. Student’s t -test P -values are shown ( n =3). Error bars: s.d. ( c ) Immunoblots of TWF1 (green band, top panel), VIM (green band, middle panel), SNAI2 (green band, bottom panel) and β-actin (red band, top panel) with protein lysates of MDA-MB-231 cells 36 h after transfections of mock control, scrambled (Scr) and oligo miRNA-30c, respectively. ( d ) Effects of miR-30c on cell morphology and F-actin. Top panels: images of MDA-MB-231 cells after miR-30c transfections. Top left panels: bright field (BF) images of cells (X200, black scale bars, 10 μm). Top right panels: fluorescent images (X1,000, white scale bars, 5 μm) with F-actin staining (green) and DAPI staining of DNA (blue). Bottom histogram: percentage of round cells counted in two groups, scrambled and 30c-transfected cells ( n =4, counting 4 replicates of 100–150 cells). Cells were collected 36 h after transfections of scramble control (top) or miR-30c oligos (bottom). Student’s t -test P =0.043. Error bars: s.d. ( e ) Luciferase activity assays of Hek293T cells co-transfected with miR-30c (or scrambled control, scr) and the luciferase vector containing wild-type (WT) or mutated (mt) 3′UTR of TWF1. Mt1, 2, 3 are mutants with G/C converted to T in individual predicted binding site 1, 2, or 3, and mt123 contains all three mutated sites (see Supplementary Fig. S3 ). Student’s t -test P =0.0001 for WT or mt2, comparing 30c with scr control ( n =5). Error bars: s.d. Full size image The function of TWF1 as a regulator of drug sensitivity was previously revealed by in vivo RNA interference screening in a lymphoma model, along with other regulators of actin dynamics, such as Rac2 [12] . TWF1 is a conserved actin-binding protein with two actin depolymerizing factor homology (ADF-H) domains [16] and belongs to the ADF-H family along with ADF/cofilin, Abp1/drebrin, coactosin and glia maturation factor [17] . It regulates diverse morphological and motile processes by both sequestering ADP-actin monomers and capping filament barbed ends [18] , [19] . We hypothesized that TWF1 is an important target of miR-30c by linking drug resistance to actin-based cytoskeletal organization, such as the stress fibre F-actin, an EMT marker. To address this hypothesis, we performed experimental validation analyses. Inhibition of TWF1 expression by miR-30c was confirmed in MDA-MB-231 cells by real-time PCR and western blots ( Fig. 3b ). In addition, transient transfection of an anti-miR-30c inhibitor increased TWF1 expression in these breast cancer cells ( Fig. 3b ). We also observed inhibitory effects of miR-30c on the EMT markers VIM and SNAI2 at protein levels compared with the scrambled miRNA control or a mock transfection control of MDA-MB-231 cells ( Fig. 3c ). Accordingly, elevated miR-30c promoted a round epithelial cell phenotype and reduced the stress fibre F-actin formation in MDA-MB-231 cells ( Fig. 3d ; large images in Supplementary Fig. S4 ). Further analyses and quantitative counting of stained vinculin revealed a reduction in focal adhesions, which further validated the effect of miR-30c on F-actin dynamics ( Supplementary Fig. S5a,b ). We then investigated whether TWF1 is a direct target of miR-30c. The functional interaction between miR-30 and the 3′UTR of TWF1 was examined in luciferase assays in HEK293T cells. Compared with the scrambled control, co-transfected miR-30c suppressed the expression of the luciferase gene, which was located upstream of the wild-type 3′UTR of TWF1 ( Fig. 3e ; see also Supplementary Fig. S6 ). Mutation of all three predicted recognition sites within the 3′UTR of TWF1 ( Supplementary Fig. S6 ) abolished the inhibitory effect of miR-30c on luciferase activity ( Fig. 3e ). These data indicate that the inhibitory function of miR-30c on the target gene requires interaction with the predicted binding sites. TWF1 is important in regulating chemoresistance and EMT To determine the importance of TWF1 in miR-30c-regulated drug resistance, we performed functional rescue assays by co-transfecting 3′UTR-deficient TWF1 cDNA and miR-30c in MDA-MB-231 cells. Although miR-30c expression induced inhibitory effects on chemoresistance, recombinantly expressed TWF1 (resistant to miR-30 inhibition) reversed miR-30c-mediated sensitivity of the cancer cells to doxorubicin and paclitaxel ( Fig. 4a ). 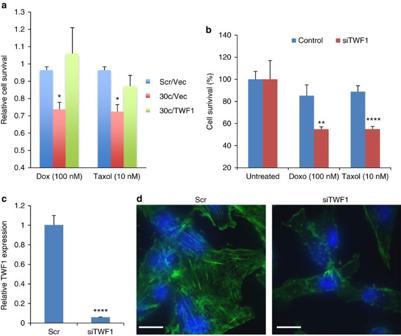Figure 4: TWF1 is required for miR-30c functions. (a) Overexpression of TWF1 reversed the chemo response sensitized by miR-30c in MDA-MB-231 cells upon doxorubicin (Doxo) or paclitaxel (Taxol) treatments. Student’st-testP=0.01 (Doxo) and 0.02 (Taxol), when comparing 30c/Vec with 30c/TWF1 (n=5). Error bars: s.d. (b) Knockdown of TWF1 by a transient transfection of siRNAs of TWF1 (siTWF1) mimicked the miR-30c overexpression to enhance the cytotoxicity of doxorubicin (Doxo) and paclitaxel (Taxol) in MDA-MB-231 cells. **P=0.0049, ****P=4.77E-05 (n=5) by a Student’st-test. Error bars: s.d. (c) Relative expression levels of TWF1 upon siRNA transfections, measured by real-time PCR (BD Taqman assays). Student’st-testP=7.31E-05 (n=3). Error bars: s.d. (d) Images of F-actin staining of MDA-MB-231 cells inhibited by siTWF1 knockdowns, compared with scrambled control (Scr) (X1,000, green for F-actin staining and blue for DAPI staining), white scale bars, 5 μm. Cells were collected 36 h after transfections. Figure 4: TWF1 is required for miR-30c functions. ( a ) Overexpression of TWF1 reversed the chemo response sensitized by miR-30c in MDA-MB-231 cells upon doxorubicin (Doxo) or paclitaxel (Taxol) treatments. Student’s t -test P =0.01 (Doxo) and 0.02 (Taxol), when comparing 30c/Vec with 30c/TWF1 ( n =5). Error bars: s.d. ( b ) Knockdown of TWF1 by a transient transfection of siRNAs of TWF1 (siTWF1) mimicked the miR-30c overexpression to enhance the cytotoxicity of doxorubicin (Doxo) and paclitaxel (Taxol) in MDA-MB-231 cells. ** P =0.0049, **** P =4.77E-05 ( n =5) by a Student’s t -test. Error bars: s.d. ( c ) Relative expression levels of TWF1 upon siRNA transfections, measured by real-time PCR (BD Taqman assays). Student’s t -test P =7.31E-05 ( n =3). Error bars: s.d. ( d ) Images of F-actin staining of MDA-MB-231 cells inhibited by siTWF1 knockdowns, compared with scrambled control (Scr) (X1,000, green for F-actin staining and blue for DAPI staining), white scale bars, 5 μm. Cells were collected 36 h after transfections. Full size image Equally important, knockdown of TWF1 by short interfering RNAs (siRNAs) copied the phenotype of high miR-30c levels by sensitizing breast tumour cells to chemotherapeutic agents doxorubicin and paclitaxel at 100 and 10 nM treatment doses, respectively ( Fig. 4b ). We further investigated the effect of TWF1 knockdown on F-actin formation in MDA-MB-231 cells. Notably, siRNAs of TWF1 dramatically inhibited F-actin organization, reduced vinculin-stained focal adhesions and promoted the mesenchymal-to-epithelial transition with a round cell shape ( Fig. 4d ; see also Supplementary Figs S4 and S5a,b ). In addition to TWF1, VIM is another EMT-related cytoskeleton gene that is inhibited by miR-30c, as shown by microarray and western blot analyses ( Fig. 3a ). Overexpression of VIM reversed the drug sensitivity caused by miR-30c ( Supplementary Fig. S7a ), suggesting that VIM is an important target of miR-30c and may partially overlap with the effect of TWF1 in regulating drug resistance. However, knockdown of VIM is not sufficient to mimic the functions of miR-30c or increase drug sensitivity ( Supplementary Fig. S7b ). IL-11 is a downstream target of miR-30c and TWF1 Interleukins (ILs) and cytokines, including IL-6 family members, have been shown to contribute to drug resistance in breast cancer and other cancers [20] , [21] , [22] , [23] . On the basis of significance analysis of microarrays, we observed that miR-30c suppressed expression of IL-11, one of the IL-6 family members, in breast cancer cells ( Fig. 3a ; see also Supplementary Data 1 ). The specific regulation of IL-11 expression by miR-30c was validated by real-time PCR analyses, demonstrating both an inhibitory effect of miR-30c oligos and a promoting effect of anti-miR-30c on IL-11 expression in MDA-MB-231 cells ( Fig. 5a ). 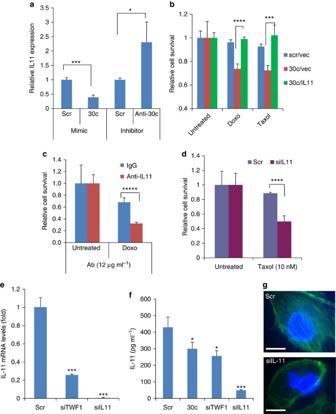Figure 5: IL-11 as a downstream target of TWF1. (a) Relative IL-11 expression levels measured by real-time PCR analyses. The miR-30c oligos (mimic) downregulated IL-11 expression, whereas the anti-miR-30c inhibitor upregulated IL-11 expression in MDA-MB-231 cells after 36 h of transfections, compared with the scrambled control (Scr). *P=0.03299, ***P=0.00052 (n=3) by a Student’st-test. Error bars: s.d. (b) Overexpression of IL-11 reversed miR-30c-mediated sensitivity of MDA-MD-231 cells to doxorubicin (Doxo) and paclitaxel (Taxol) (n=6). Student’st-testP=2.8E-05 (Doxo) and 1.1E-04 (Taxol), when comparing 30c/vector with 30c/IL-11. Error bars: s.d. (c) Survival of MDA-MB-231 cells incubated with the goat IgG control or a neutralizing antibody to human IL-11 (12 μg ml−1), upon 72 h exposure to 100 nM doxorubicin (Doxo). *****P=4.24E-06 by a Student’st-test (n=6). Error bars: s.d. (d) Knockdown of IL-11 by siRNAs sensitized cytotoxicity of MDA-MB-231 cells to 72-h treatment of paclitaxel (Taxol, 10 nM). ****P=3.0E-05 by Student’st-test (n=6). Error bars: s.d. (e) Reduction of IL-11 mRNA expression upon gene knockdowns of siTWF1 and siIL-11, compared with the scrambled control (Scr) (n=3), measured by real-time PCR. ***P=0.0009 (siTWF1) and 0.0003 (siIL-11) by a Student’st-test. Error bars: s.d. (f) IL-11 levels detected in the cultured media of MDA-231 cells, upon transfections with scrambled, miR-30c and siRNAs for TWF1 or IL-11 (n=4). Student’st-testP=0.0381 (30c), 0.0329 (siTWF1), 0.0007 (siIL11) compared to the scrambled control (Scr). Error bars: s.d. (g) Images of F-actin staining of MDA-MB-231 cells, transfected with siRNAs of IL-11 and scrambled control (Scr) (X1,000, green for F-actin staining and blue for DAPI staining), white scale bars, 5 μm. Cells were collected 36 h after transfections. Figure 5: IL-11 as a downstream target of TWF1. ( a ) Relative IL-11 expression levels measured by real-time PCR analyses. The miR-30c oligos (mimic) downregulated IL-11 expression, whereas the anti-miR-30c inhibitor upregulated IL-11 expression in MDA-MB-231 cells after 36 h of transfections, compared with the scrambled control (Scr). * P =0.03299, *** P =0.00052 ( n =3) by a Student’s t -test. Error bars: s.d. ( b ) Overexpression of IL-11 reversed miR-30c-mediated sensitivity of MDA-MD-231 cells to doxorubicin (Doxo) and paclitaxel (Taxol) ( n =6). Student’s t -test P =2.8E-05 (Doxo) and 1.1E-04 (Taxol), when comparing 30c/vector with 30c/IL-11. Error bars: s.d. ( c ) Survival of MDA-MB-231 cells incubated with the goat IgG control or a neutralizing antibody to human IL-11 (12 μg ml −1 ), upon 72 h exposure to 100 nM doxorubicin (Doxo). ***** P =4.24E-06 by a Student’s t -test ( n =6). Error bars: s.d. ( d ) Knockdown of IL-11 by siRNAs sensitized cytotoxicity of MDA-MB-231 cells to 72-h treatment of paclitaxel (Taxol, 10 nM). **** P =3.0E-05 by Student’s t -test ( n =6). Error bars: s.d. ( e ) Reduction of IL-11 mRNA expression upon gene knockdowns of siTWF1 and siIL-11, compared with the scrambled control (Scr) ( n =3), measured by real-time PCR. *** P =0.0009 (siTWF1) and 0.0003 (siIL-11) by a Student’s t -test. Error bars: s.d. ( f ) IL-11 levels detected in the cultured media of MDA-231 cells, upon transfections with scrambled, miR-30c and siRNAs for TWF1 or IL-11 ( n =4). Student’s t -test P =0.0381 (30c), 0.0329 (siTWF1), 0.0007 (siIL11) compared to the scrambled control (Scr). Error bars: s.d. ( g ) Images of F-actin staining of MDA-MB-231 cells, transfected with siRNAs of IL-11 and scrambled control (Scr) (X1,000, green for F-actin staining and blue for DAPI staining), white scale bars, 5 μm. Cells were collected 36 h after transfections. Full size image To determine the role of IL-11 in the miR-30c pathway, we also performed functional rescue studies by modulating IL-11 expression levels and functions. Overexpression of IL-11 reversed miR-30c-mediated drug sensitivity of MDA-MB-231 cells to doxorubicin and paclitaxel ( Fig. 5b ). In addition, we examined the effect of a neutralizing antibody to human IL-11 on drug response of MDA-MB-231 cells. The anti-IL-11 IgG added to culture media indeed copied the function of miR-30c by sensitizing cells to the doxorubicin treatment ( Fig. 5c ), suggesting that the secreted form of IL-11 has a role in mediating drug resistance. Similarly, siRNA-mediated knockdown of IL-11 sensitized the response of MDA-MB-231 cells to paclitaxel ( Fig. 5d ). On the basis of Geneset2miRNA target gene predictions, IL-11 was not on the list of predicted direct targets of miR-30 ( Supplementary Table S6 ), suggesting that it may be a secondary target of miR-30c. We therefore explored the regulatory link between miR-30c and IL-11. As actin affects the activity of myocardin-related transcription factors (MRTFs) and serum response factor, which regulate expression of IL-11 ( [24] ), we hypothesized that TWF1, also an upstream regulator of actin dynamics, regulates IL-11 expression. We therefore examined the effect of modulated TWF1 on IL-11. As anticipated, siRNA-mediated knockdown of TWF1 inhibited IL-11 mRNA and protein expression in MDA-MB-231 cells, similar to the effect of miR-30c on IL-11 ( Fig. 5e ). These data suggest that IL-11 is an important target of TWF1 in the miR-30c signalling pathway, which regulates breast cancer chemoresistance. We then examined whether IL-11 also regulated F-actin formation. Indeed, knockdown of IL-11 displayed a mesenchymal-to-epithelial transition phenotype very similar to that of miR-30c or knockdown of TWF1, as demonstrated both by F-actin staining and by counting of vinculin-stained focal adhesions ( Fig. 5g ; see also Supplementary Figs S4 and S5a,b ). miR-30c regulates chemoresistance in vivo To validate the role of miR-30c as a regulator of breast tumour progression in vivo , we examined the effects of miR-30c precursor expression on chemoresistance, using triple negative human breast tumour xenograft models generated from breast tumour-initiating cells (BTICs) [25] . To facilitate the monitoring of miR-expressing cells in vivo , we cloned the miR-30c precursor into a lentiviral vector (pFU-miR-30c-PGK-L2G) that co-expresses the dual-reporter luciferase gene Luc2-eGFP ( L2G ) in transduced cells. On the basis of bioluminescence imaging following orthotopic transplantation, miR-30c precursor expression did not alter BTIC-mediated tumour growth in vivo ( Supplementary Fig. S8a,b ). At a dose of 1 mg kg −1 , doxorubicin did not inhibit tumour growth mediated by BTICs expressing the empty L2G vector control, but did significantly inhibit the growth of L2G-30c-expressing tumour cells ( n =20, P ≤0.00001; Fig. 6a ). This result indicates that expression of the miR-30c precursor reversed the resistance of the human breast tumour model to doxorubicin treatment in vivo . 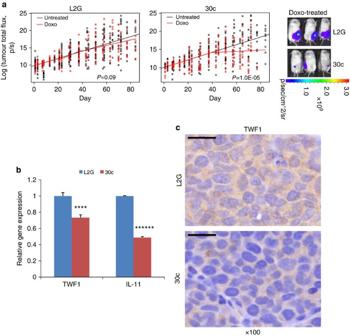Figure 6: miR-30c regulates chemoresistance of breast tumourin vivo. (a) Doxorubicin treatment response (log-transformed bioluminescence signals) of implanted CD44+human breast tumour cells expressing L2G vector control (left panel,n=40) and miR-30c (middle panel,n=40). The right panel pictures are representative bioluminescence images of treated mice: L2G control (top) and 30c-overexpressed (bottom). Doxorubicin (or PBS vehicle control for untreated) was given intraperitoneally at 1 mg kg−1to treated mice on day 20 and day 39. In the vector control mice (top panel), doxorubicin (red) did not significantly inhibit tumour growth (slope change after treatmentP>0.05, R statistical package analysis) compared to the untreated group (black). In the miR-30c precursor overexpression group (bottom panel), doxorubicin (red) inhibited tumour growth (slope changeP-values shown, R model analysis). (b) TWF1 and IL-11 mRNA levels inhibited by pFU-PGK-L2G mediated miR-30c precursor expression in xenograft breast tumour cells (sorted from human-in-mouse tumoursin vivo), measured by real-time PCR. Student’st-testP=0.0001 (TWF1) and 1.04E-07 (IL-11) (n=3). Error bars: s.d. (c) Reduced immunohistochemistry staining against human TWF1 in one of three representative 30c-overexpressing primary breast tumour sections, compared with L2G-vector-transduced tumour sections (X100). Scale bars, 20 μm in both images. Figure 6: miR-30c regulates chemoresistance of breast tumour in vivo . ( a ) Doxorubicin treatment response (log-transformed bioluminescence signals) of implanted CD44 + human breast tumour cells expressing L2G vector control (left panel, n =40) and miR-30c (middle panel, n =40). The right panel pictures are representative bioluminescence images of treated mice: L2G control (top) and 30c-overexpressed (bottom). Doxorubicin (or PBS vehicle control for untreated) was given intraperitoneally at 1 mg kg −1 to treated mice on day 20 and day 39. In the vector control mice (top panel), doxorubicin (red) did not significantly inhibit tumour growth (slope change after treatment P >0.05, R statistical package analysis) compared to the untreated group (black). In the miR-30c precursor overexpression group (bottom panel), doxorubicin (red) inhibited tumour growth (slope change P -values shown, R model analysis). ( b ) TWF1 and IL-11 mRNA levels inhibited by pFU-PGK-L2G mediated miR-30c precursor expression in xenograft breast tumour cells (sorted from human-in-mouse tumours in vivo ), measured by real-time PCR. Student’s t -test P =0.0001 (TWF1) and 1.04E-07 (IL-11) ( n =3). Error bars: s.d. ( c ) Reduced immunohistochemistry staining against human TWF1 in one of three representative 30c-overexpressing primary breast tumour sections, compared with L2G-vector-transduced tumour sections (X100). Scale bars, 20 μm in both images. Full size image To examine the functional relevance of downstream signalling pathways in vivo , we measured the expression levels of target genes in sorted breast cancer cells. Compared with vector L2G-transduced cancer cells, inhibition of TWF1 and IL-11 expression was confirmed in sorted miR-30c-expressing human breast tumour cells isolated from tumour models in vivo ( Fig. 6b ). Furthermore, the reduction of TWF1 expression at the protein level was confirmed in miR-30c-expressing tumours by immunohistochemical staining ( Fig. 6c ). These studies convincingly demonstrated that miR-30c regulates the downstream TWF1 and IL-11 targets and signalling pathways in vivo . GATA3 regulates miR-30c expression in breast cancer To investigate mechanisms by which miR-30c is downregulated in group one breast tumours, we examined possible regulation by transcription factors (TFs). JASPAR online analysis ( jaspar.genereg.net ) [26] identified predicted TF binding sites in the putative miR-30c promoter regions, including GATA3 binding sites ( Supplementary Table S7 ). TF–miRNA association analyses showed that GATA3 mRNA expression levels correlated with miR-30c expression levels in breast tumours (UC set, n =44, P =0.023; Fig. 7a ); a separate Oxford breast tumour data set showed a similar correlation [6] ( n =210, P <0.001; Fig. 7a ). In addition, forced expression of wild-type GATA3 induced a significant increase (eight- to ninefold) of miR-30c expression in GATA3-deficient MDA-MB-231 breast cancer cells ( n =6, P =1.95E-08; Fig. 7b ). These data indicate that GATA3 regulates miR-30c in breast tumours. 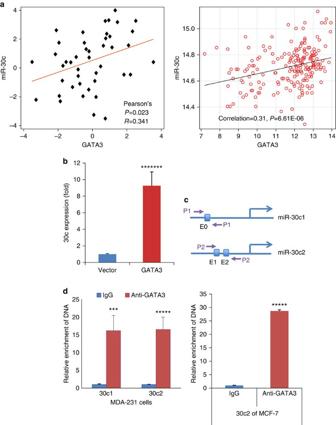Figure 7: GATA3 regulation of miR-30c. (a) Scatter plots of GATA3 expression and miR-30c levels in UC set breast tumours (n=44,P=0.023, R=0.341; left panel) and Oxford breast tumour sets (GSE22220 and GSE22216;n=210,P=0.0005, Pearson’s correlation=0.31) (right panel). Linear regression analyses were performed between miRNA expression and GATA3 levels after log2 transformation. Plots were drawn using the scatterplot function found in the Car package (http://cran.r-project.org). (b) Induced expression of miR-30c (Student’st-testP=1.95E-08,n=5) by ectopic GATA3 in MDA-MB-231 breast cancer cells, measured by real-time PCR, compared with the vector control. Error bars: s.d. (c) 3 kb promoter regions ofhsa-miR-30c1and30c2with predicted GATA3-binding elements (E0 for30c1, E1 and E2 for30c2). PCR primers were designed to amplify the regions flanking E0 (P1) or both E1 and E2 (P2). (d) Left panel: themiR-30cpromoter regions of30c1and30c2enriched by GATA3 antibody-mediated ChIP with GATA3-overexpressing MDA-MB-231 lysates, detected by real-time PCR using primers P1 and P2, respectively. Right panel: themiR-30c2promoter enriched by GATA3 antibody-mediated ChIP with MCF-7, detected by real-time PCR with P2 primers. Student’st-testP=0.0004 (30c1) and 3.59E-06 (30c2) for MDA-MB-231 cells and 5.23E-06 (30c2) for MCF-7 cells, respectively (n=6). Error bars: s.d. Figure 7: GATA3 regulation of miR-30c. ( a ) Scatter plots of GATA3 expression and miR-30c levels in UC set breast tumours ( n =44, P =0.023, R=0.341; left panel) and Oxford breast tumour sets (GSE22220 and GSE22216; n =210, P =0.0005, Pearson’s correlation=0.31) (right panel). Linear regression analyses were performed between miRNA expression and GATA3 levels after log2 transformation. Plots were drawn using the scatterplot function found in the Car package ( http://cran.r-project.org ). ( b ) Induced expression of miR-30c (Student’s t -test P =1.95E-08, n =5) by ectopic GATA3 in MDA-MB-231 breast cancer cells, measured by real-time PCR, compared with the vector control. Error bars: s.d. ( c ) 3 kb promoter regions of hsa-miR-30c1 and 30c2 with predicted GATA3-binding elements (E0 for 30c1 , E1 and E2 for 30c2 ). PCR primers were designed to amplify the regions flanking E0 (P1) or both E1 and E2 (P2). ( d ) Left panel: the miR-30c promoter regions of 30c1 and 30c2 enriched by GATA3 antibody-mediated ChIP with GATA3-overexpressing MDA-MB-231 lysates, detected by real-time PCR using primers P1 and P2, respectively. Right panel: the miR-30c2 promoter enriched by GATA3 antibody-mediated ChIP with MCF-7, detected by real-time PCR with P2 primers. Student’s t -test P =0.0004 (30c1) and 3.59E-06 (30c2) for MDA-MB-231 cells and 5.23E-06 (30c2) for MCF-7 cells, respectively ( n =6). Error bars: s.d. Full size image To determine whether GATA3 binds directly to the miR-30c promoters ( 30c1 and 30c2 ), we performed chromatin immunoprecipitation (ChIP) assays with anti-GATA3 antibodies (Santa Cruz) using lysates of MCF-7 cells that express endogenous GATA3 and lysates of MDA-MB-231 cells that contain ectopically expressed GATA3. By ChIP and real-time PCR analyses, we observed an interaction between GATA3 with the 30c2 promoter, which contains two predicted binding elements in both cell lines and an interaction between GATA3 and the 30c1 promoter in MDA-MB-231 cells ( Fig. 7c-d ). These data collectively demonstrate that GATA3 transcriptionally regulates miR-30c expression in breast tumour cells. The importance of miR-30c in a clinically relevant pathway To validate the importance of the miR-30c signalling transduction pathway in clinical tumours, we examined the association of miR-30c with its target genes. On the basis of the Oxford breast tumour data set [6] with combined mRNA and miRNA expression profiles, we observed a negative correlation between miR-30c and IL-11 expression ( Fig. 8a , n =210, P =0.005). In the recently completed Breast Cancer data set in The Cancer Genome Atlas (TCGA) [27] , we also verified inverse correlations between miR-30c and TWF1, and between miR-30c and IL-11 ( Supplementary Table S8 , n =521, P =0.0077 and 0.0002, respectively). 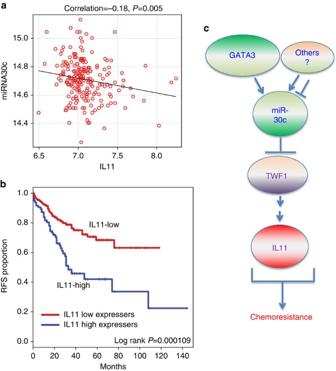Figure 8: Clinical relevance of the miR-30c signalling pathway. (a) Scatter plots between IL-11 single gene expression and the expression of miR-30c in breast cancer data set with combined expression profiles of mRNA GSE22220 and miRNA GSE22216 (n=210). Pearson’s correlation was estimated (P=0.005). (b) Survival outcomes of IL-11 gene expression in primary breast cancers in the UNC337 publicly available microarray data set8. Relapse-free survival KM plots were based on IL-11 gene expression and median gene expression was used to define low and high expressers (P=0.000109,n=337). (c) Signalling pathway scheme GATA3-miR30-TWF1-IL-11 regulation of breast cancer chemo-resistance. Figure 8: Clinical relevance of the miR-30c signalling pathway. ( a ) Scatter plots between IL-11 single gene expression and the expression of miR-30c in breast cancer data set with combined expression profiles of mRNA GSE22220 and miRNA GSE22216 ( n =210). Pearson’s correlation was estimated ( P =0.005). ( b ) Survival outcomes of IL-11 gene expression in primary breast cancers in the UNC337 publicly available microarray data set [8] . Relapse-free survival KM plots were based on IL-11 gene expression and median gene expression was used to define low and high expressers ( P =0.000109, n =337). ( c ) Signalling pathway scheme GATA3-miR30-TWF1-IL-11 regulation of breast cancer chemo-resistance. Full size image In addition, relapse-free analysis with and without adjustment for nodal status, ER, grade, treatment and tumour stage demonstrated that IL-11 is strongly associated with clinical outcome in three independent breast tumour sets (UNC337, Oxford tumour set and UC tumour set) for which IL-11 is a poor prognostic marker ( Fig. 8b ; see also Supplementary Table S9 ). The above data suggest a signalling network ( Fig. 8c ) that links miR-30c with its upstream TF GATA3 and with its downstream targets TWF1 and IL-11, and demonstrates the clinical importance of the miR-30c-regulated pathway in human breast cancer. Our results implicate miR-30c as a phenotypic regulator of chemoresistance. Although our studies focus on the role of miR-30c as a regulator of chemotherapy response in breast tumours, miR-30c expression has been correlated with endocrine therapy resistance, which is often linked to chemotherapy resistance in advanced ER-positive breast cancer [9] . EMT (VIM expression) has been linked with breast tumour-initiating cell resistance to endocrine therapy and chemotherapy [2] . Our data demonstrate that miR-30c regulates breast cancer chemoresistance and EMT (F-actin formation) by direct targeting of the cytoskeleton gene TWF1 , as well as by indirect targeting of the cytokine IL-11. Although TWF1 is known to have a significant role in regulating cancer cell chemoresistance [12] , the underlying mechanisms are not known. We have identified IL-11 as a relevant downstream target of TWF1 and demonstrated novel roles for TWF1 and IL-11 in regulating F-actin formation, an EMT marker. IL-11 belongs to the IL-6 family, which have been associated with drug sensitivity in various cancers and epithelial tissues [21] , [23] , [28] . Interestingly, TWF1 regulates the expression of IL-11 at both the mRNA and protein levels, although the detailed mechanisms remain to be elucidated. As TWF1 is an actin-binding protein, it is likely that TWF1 regulates IL-11 through sequestering actin monomers, thereby reducing the free actin monomer pool. A reduced actin monomer pool could release actin-bound MRTFs, especially MRTFA, from trapping, thereby activating MRTFs for nuclear translocation [24] , [29] . Activated MRTF binds to and assists serum response factor to transactivate IL-11 transcription, as MRTFA −/− cells display reduced IL-11 expression levels [24] . It is of great interest to explore regulatory mechanisms of aberrantly expressed miRNAs in breast cancer. Our studies have identified GATA3 as a transcriptional regulator of miR-30c. GATA3 has an important role in both normal mammary development and breast tumour differentiation, and its expression correlates with luminal epithelial phenotype and ER status [30] , [31] , [32] . MiR-30c promoter analyses also show predicted binding sites for other TFs (for example, YY1 and BRCA1) that may contribute to the regulation of miR-30c expression. However, we did not observe significant correlation between YY1 and BRCA1 expression and miR-30c in the UC tumour set (data not shown). In addition to transcriptional regulation, other mechanisms can contribute to deregulated miRNA expression, such as chromatin deletions/amplifications, translocations, promoter silencing and deficient post-transcriptional processing. In a separate study, we observed copy number variation at chromatin regions containing miR -30c1 and miR-30c2 genes (Nwachukwu et al . (2012), submitted). In conclusion, we have identified a novel miRNA-mediated pathway that regulates chemoresistance in breast cancer. The components of this pathway, including GATA3, miR-30c, TWF1 and IL-11, represent attractive targets for developing new therapeutic strategies in the management of breast cancer. All experiments were performed under the approval of the Institutional Biosafety Committee, Institutional Review Board and the Administrative Panel on Laboratory Animal Care of University of Chicago. All experiments had multiple replicates. Breast tumour arrays and subtypes Total RNAs were extracted from frozen tissues and cultured cells for DNA microarrays (Agilent Technologies) as described [34] . All microarray and patient clinical data are available at UNC Microarray Database ( https://genome.unc.edu ) and in the Gene Expression Omnibus (GEO) under accession number GSE22049 (clinical tumour/tissues) and GSE32617 (MDA-MB-231 cells). Breast tumours subtype determination was based on gene expression (PAM50 5-subtype predictor [7] and claudin-low predictor [35] ), as well as immunohistochemical staining for ER, PR, HER2, EGFR, CK5/6, and CK8/18 [36] . miRNA expression arrays The miRNA arrays, deposited in GEO under accession number GSE39543 , were performed for frozen primary breast specimens ( n =51) by Exiqon (Woburn) using the miRCURY Hy3/Hy5 power labelling kit and the miRCURY LNA Array (v.10.0; 757 human miRs). The expression values are log2 (Hy3/Hy5) ratios. Unsupervised hierarchical clustering of miRNAs was performed [34] . miRNA association tests Log2-transformed miRNA levels were used in the miR-phenotype and miR-gene association tests. Expressions of miRNAs across breast tumour subtypes were compared using analysis of variance. P -values were calculated using permutation test. For chemoresistance association analysis, AUC (the area under the survival-concentration curve) was calculated by A linear correlation test with Log 2-transformed values of AUC (or % survival) and miRNA levels were applied in the association test using R software. The correlations between genes and miRNA-30c expression were interrogated in the UC breast tumour set ( n =44) and TCGA Breast Cancer data set ( n =521 breast samples) [27] . The normalized gene (‘BRCA.exp.547.med.txt’) and miRNA (‘BRCA.780.precursor.txt’) expression matrixes were used as provided in the TCGA portal ( http://tcga-data.nci.nih.gov/docs/publications/brca_2012/ ). Pearson’s correlation coefficients were then determined between the expression of each gene and miRNA-30c (‘hsa-mir-30c.MIMAT0000244’). RNA extraction and real-time PCR Total RNAs for array analysis were extracted using Trizol (Invitrogen) and RNAeasy mini kit (Qiagen), or RNA was precipitated with isopropanol and glycogen (Invitrogen). RT–PCR for miRNAs/genes used individual miRNA/gene Taqman primers (Applied Biosystems). RNU44 and U6 primers were used for miRNA internal controls, and GAPDH for a housekeeping gene control. Vectors and cloning A lentiviral gateway vector pFU-attr-PGK-L2G was constructed based on pFU-L2G [25] , and subcloned with miRNA precursor entry clones using LR clonase II (Invitrogen). Human TWF1 cDNA was subcloned into pDEST40 (Invitrogen) from a donor vector (ORFeome collection, University of Chicago). Human IL-11 and GATA3 (transcript variant 2) expression vectors were purchased from Origene. Luciferase vector containing the 3′UTR of TWF1 was obtained from Switchgear Genomics. A site-directed mutagenesis kit (Stratagene) with appropriate primers (IDT) was used to mutate miR-30-binding sites. Cell culture and transfections Cells were maintained in DMEM (MDA-MB-231, MCF7 and Hek293T with G418) or EMEM (BT-20) with 10% fetal bovine serum±1% Penicillin-Streptomycin. miRNAs (Dharmacon, negative control number 4), anti-miRNAs (Exiqon, negative control A) and siRNAs (pooled; Dharmacon) were transfected using Dharmafect (Dharmacon) at 100 nM (MDA-MB-231) or 50 nM (BT-20, Hek293T), and repeated on the following day. The 3′UTR luciferase vectors and cDNA vectors were transfected using Fugene (Roche-Promega). For target gene rescue experiments, cells were transfected twice with cDNA vectors after two 6-h miRNA transfections. Cell growth assays Transfected cells were plated in phenol red free media. Next day, calcein AM (Invitrogen) was added to the wells at 4 μg μl −1 and incubated for an hour at 37 °C. Plates were read at 485/535 nM on the Wallac 1420 plate reader (Perkin Elmer). Western blot Cells were collected 48 h after transfections, lysed and sonicated in RIPA buffer. Protein (100 μg) was loaded onto 4–20% gradient gels for immunoblots with antibodies to TWF1 (Genetex, GTX11439), VIM (Abcam, ab61780), SNAI2 (Cell Signalling, number 9585) and β-actin (Sigma-Aldrich, AC-15). Blots were read on Odyssey (Li-Cor). IL protein level measurement Cell culture media were collected 36 h post transfections. IL protein levels in the supernatants were measured using human cytokine magnetic beads and detection kit (Millipore) and read by Bioplex (BioRad). Luciferase assay Hek293T cells were transfected with miRNAs followed by transfection overnight with 3′UTR luciferase and control renilla vectors (Promega). Cells were lysed 48 h later and measured using a dual luciferase kit (Promega). The luciferase signal was normalized to renilla. Drugs, cytotoxicity and apoptosis Paclitaxel and doxorubicin were obtained from either Chemopharmacy at the University of Chicago or Sigma. Breast cancer cells (ATCC) were treated for 72 h with doxorubicin (0–1,000 nM) and paclitaxel (0–10 nM). Cytotoxicity was measured using AlamarBlue (Invitrogen). Survival of cells were measured using cell titre blue (Promega) after 72 h (MDA-MB-231) or 48 h (BT-20) treatment. Anti-IL-11 neutralizing antibody (R&D Systems) was added at 12 μg ml −1 before treatment. One day post transfection, cells were exposed to doxorubicin (100 nM) and paclitaxel (10 nM) for 24 h, and collected for fixation in 70% ethanol and staining with propidium iodide (Sigma). DNA content was analysed using BD LSRII flow cytometer. Immunofluorescence, histology and microscope Transfected cells were plated on microscope slides (Millipore) for F-actin and focal adhesion staining. Cells were fixed in 4% paraformaldehyde/PBS, washed and stained with fluorescent phalloidin (Invitrogen F432) and SlowFade Gold antifade reagent with DAPI (Invitrogen) or anti-vinculin (ab18058, Abcam). Secondary antibody was anti-mouse Texas Red (T-862, Invitrogen). Cell images were taken using Axiovert 100tv (fluorescent), Axiovert 200 M (phase contrast; Zeiss) or Olympus spinning disc confocal microscope. Focal adhesions were quantified using ImageJ software with 50 cells counted per well. Tumour and lung samples were fixed in 10% neutral buffered formalin, embedded and sectioned. Immunohistochemical staining was performed using green fluorescent protein(Cell Signalling, number 2956) and hTWF1 (GeneTex, GTX11439) antibodies at the Histology facility. Images were taken by Pannoramic Scan Whole Slide Scanner (CRi, Cambridge Research and Instrumentation). Chromatin immunoprecipitation (ChIP) GATA3 antibodies (Santa Cruz, catalogue number 268 for MDA-MB-231 cells, catalogue number 269 for MCF-7 cells) were used for ChIP according to the EZ ChIP Chromatin Immunoprecipitation Kit (Millipore Upstate Cell Signalling Solutions, catalogue number 17–371). DNA was purified using a phenol–chloroform extraction and precipitated by ethanol and glycogen. DNA was quantified using Fast SYBR Green Master Mix (Applied Biosystems). The sequences of 30c1-P1 primers: 5′-TGTGGGCTGCCTGCTGAATACAC-3′ and 5′-AGCAAGAGTGAACTGCTGCCTCCT-3′; and 30c2-P2 primers: 5′-TTTGGAAGGGGTGGGCAGTGAAGA-3′ and 5′-ACTGACATGGTCATCCCACTTGC-3′. Tumour cell isolation and flow cytometer analysis Xenograft tumours were collected from mice with 1,800 units collagenase III (Worthington) and 100 Kunitz units DNase I (Sigma) as described [25] . Dissociated tumour cells were stained with CD44-APC, H2Kd-biotin and strepavidin-PE-cy7 (BD), and DAPI in HBSS/2% fetal bovine serum for further flow analysis or sorting on FacsAriaII (BD). Lentivirus production and transduction Second-generation packaging vectors (VPR and VSVG) [25] were used to produce miRNA precursor lentiviruses, and third-generation packaging vectors (pRSV-rev, VSVG and pMDLg/RRE) for other lentiviruses. Viable CD44+ breast cancer cells were isolated from TN1 xenograft tumours [25] and transduced with lentiviruses at 10 or 20 multiplicities of infection (MOI 10 or 20). Tumour transplantation and chemotherapy in mice Tumour cells were mixed 1:1 with Matrigel (BD) and transplanted into NOD/SCID mouse mammary fad pads (both left 4th and right 4th mammary fat pads) [25] , with a cohort of 10–20 mice per sample. Doxorubicin was injected intraperitoneally at 1 mg kg −1 of mouse weight on day 20 and day 39 post implantation. Tumour growth was measured weekly by bioluminescence imaging. Bioluminescence imaging As described [25] , bioluminescence images were acquired after D-luciferin (Biosynth AG) injection to mice (intraperitoneally, 100 μl at 30 mg ml −1 per mouse) or incubation (300 μg ml −1 ) with dissected lungs and tissues, using the IVIS Spectrum system (Caliper Life Sciences). Data was analysed using LivingImage 4.0 Software (Caliper Life Sciences) and expressed as total photon flux. Statistical Analysis If not specified otherwise, a Student’s t -test was used to evaluate significance, P -values and s.d. For animal studies, tumour growth curves were analysed using a linear mixed model in R software [37] , with the tumour volume (bioluminescence signals) or its fold change as a response variable. Lung metastases were analysed using Wilcoxon rank sum test. Log transformation was taken on both tumour volume and its fold change. For predictors, time, group indicator (vector control versus miRNA overexpression, treated versus untreated) and their interactions were considered initially; then, non-significant ones were dropped later and only significant variables were kept in the final models. As two tumours were planted and observed from each mouse, mouse ID (ear tag number) was included in the model as random effect. To allow autocorrelation among the tumour size measurements from the same mouse, AR (1) (autoregressive model of order 1) was added to the error term. Accession codes: Microarray and patient clinical data have been deposited in the Gene Expression Omnibus under accession codes GSE22049 (clinical tumour/tissues), GSE32617 (MDA-MB-231 cells) and GSE39543 (frozen primary breast specimens). How to cite this article: Bockhorn, J. et al ., MicroRNA-30c inhibits human breast tumour chemotherapy resistance by regulating TWF1 and IL-11. Nat. Commun. 4:1393 doi: 10.1038/ncomms2393 (2013).